Wide-range and area-selective threshold voltage tunability in ultrathin indium oxide transistors The scaling of transistors with thinner channel thicknesses has led to a surge in research on two-dimensional (2D) and quasi-2D semiconductors. However, modulating the threshold voltage ( V T ) in ultrathin transistors is challenging, as traditional doping methods are not readily applicable. In this work, we introduce a optical-thermal method, combining ultraviolet (UV) illumination and oxygen annealing, to achieve broad-range V T tunability in ultrathin In 2 O 3 . This method can achieve both positive and negative V T tuning and is reversible. The modulation of sheet carrier density, which corresponds to V T shift, is comparable to that obtained using other doping and capacitive charging techniques in other ultrathin transistors, including 2D semiconductors. With the controllability of V T , we successfully demonstrate the realization of depletion-load inverter and multi-state logic devices, as well as wafer-scale V T modulation via an automated laser system, showcasing its potential for low-power circuit design and non-von Neumann computing applications. The field-effect transistor (FET) is a fundamental component in modern electronics. The threshold voltage ( V T ) of a FET is a key parameter that determines its electronic functions, not only defining its switching modes but also scaling the supply voltage in the logic gates. In modern circuits, transistors are often tailored with different V T during the manufacturing process to enhance performance and lower power consumption. The ability to precisely control the V T of a transistor allows it to be used as a memory element, such as flash memory. In recent years, beyond-binary tunability between the “1” and “0” states has become particularly interesting in post–von Neumann applications, such as neuromorphic computation [1] , [2] , multi-state memory [3] , [4] and multiplexed sensing [5] . The capacity to finely tune V T over a wide range is crucial for these applications, as it directly impacts the storage capacity and weight precision of associated devices. It enables the development of advanced technologies that can perform complex tasks and have a wide range of applications in fields such as artificial intelligence, machine learning, and the Internet of Things (IoT). Atomically thin semiconductors, including two-dimensional and other quasi-2D materials, have shown great potential to develop beyond-silicon electronics. Indium oxide (In 2 O 3 ) recently emerged as a promising channel material for FETs as it can be thinned down to 1 nm and maintains high electron mobility beyond 100 cm 2 V –1 s –1 , showing high on-state drain current density I D > 20 A mm −1 (refs. [6] , [7] ). This advancement allows for the scaling of In 2 O 3 to align with modern technology nodes, and is expected to complement silicon-based systems for future back-end-of-line (BEOL) integration, expanding its range of applications beyond display technology. Moreover, In 2 O 3 exhibits high potential to engineer the V T as a benefit generally granted to the oxide semiconductors (OS) [8] . In modern FETs, V T is tuned during fabrication by adjusting the implanted dopant concentration or by modifying the work function of the gate. To enable dynamic control over V T , additional charge-trapped layers are required, e.g., a floating gate [9] , [10] . In OS-based FETs, V T can be tuned by various approaches such as post-fabrication thermal annealing [11] , [12] , chemical doping [13] , passivation [14] , metal decorations [15] , and incorporating a gate electrode with selected work functions [16] , etc. It is known that vacancy-related surface effects play a crucial role in altering the charge carrier density of the OS, leading to the ease of V T tunability. Even though the vacancy-related surface effects can be easily controlled, scalable V T modulation with fine control over wide ranges is still challenging. In this work, we report wide-range V T tunability in ultrathin In 2 O 3 FETs achieved via a simple optical-thermal combined method. The method involves alternating ultraviolet (UV) illumination and oxygen annealing to achieve negative and positive V T tuning, respectively. The V T of a 2 nm-thick In 2 O 3 transistor (30 nm-thick SiO 2 as the dielectric) exhibits a tunable window of 20 V with a resolution of 0.05 V, equivalent to a maximum change of sheet carrier density ( n 2D ) from 2 \(\times\) 10 10 cm −2 to 2 \(\times\) 10 12 cm −2 with a resolution of 10 9 cm −2 . Importantly, this method is an entire post-fabrication process, and the V T modulation is reversible. We show that the V T of distributed transistors in a circuit can be selectively tuned, enhancing the gain of a depletion-load inverter by an order of magnitude. Exploiting the spatial V T tunability, we show that such local control of V T can be used to pattern the V T profile in a channel of a transistor to enable multi-step transfer characteristics, advocating potential for innovative logic design and neuromorphic applications. To further demonstrate the wafer-scale practicality, we fabricated In 2 O 3 transistors on a 4-inch wafer and utilize the industry-level laser illumination system to achieve automatic large-area V T tuning for selected In 2 O 3 transistors across the entire wafer. 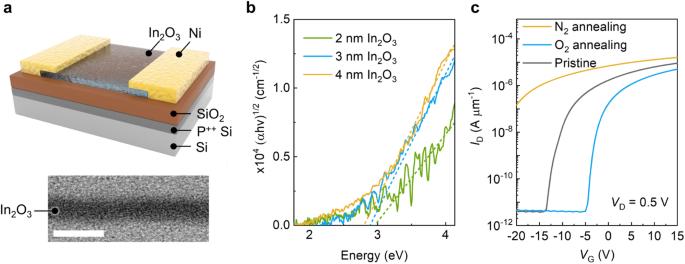Fig. 1: Device structures and high-resolution transmission electron microscopy (HRTEM) images of atomic layer deposition (ALD) deposited In2O3transistors. aSchematic of a 2 nm In2O3transistor. The inset shows the HRTEM image of the ALD-deposited ultrathin In2O3films. The scale bar is 5 nm.bTauc plot of the In2O3films as a function of film thickness. The fitting of the curve is done based on the Tauc model (α: absorption coefficient; h: Planck’s constant; ν: frequency of vibration).cTransfer curves of 2 nm In2O3transistors with channel width/length of 10/2 µm and annealed under N2and O2for 30 min at 150 °C. Note that the amounts of threshold voltage (VT) shifts are saturated after 30 minutes (ID: drain current;VD: drain voltage;VG: gate voltage). Indium has been utilized across a variety of applications (element scarcity is shown in Supplementary Table 1 ), including displays (e.g., IGZO), transparent electrodes (e.g., ITO), and solar cells (e.g., CIGS). In this study, ultrathin In 2 O 3 is employed as the channel material of a transistor, as shown schematically in Fig. 1a . The transistor is fabricated using atomic layer deposition (ALD) to form a 2–4 nm In 2 O 3 layer on p ++ Si substrates with a 30 nm-thick SiO 2 . Nickel is used as the source and drain contacts. It is important to note that the entire fabrication process is compatible with back-end-of-line (BEOL) CMOS processes, as it is carried out below the thermal budget of 300 °C (“Methods”) [17] . The high-resolution transmission electron microscopy (HRTEM; Supplementary Fig. 1 ) image reveals the amorphous nature and the atomic level uniformity of the In 2 O 3 films is confirmed by AFM (Supplementary Fig. 2 ), which effectively accounts for the minimal device-to-device variation (Supplementary Fig. 3 ). It has been shown that In 2 O 3 shows high electron mobilities even in an amorphous phase [18] . This is because the electronic property of OS is insensitive to crystallinity. Their transport is determined by the overlapping of s orbitals between neighboring metal atoms (e.g., indium) and is less affected by structural disorders [8] . The Tauc plot extracted from absorption spectra (Fig. 1b and Supplementary Fig. 4 ) shows that the bandgap of In 2 O 3 increases with decreasing channel thickness ( t ch ), from 2.7 eV ( t ch = 4 nm) to 3 eV ( t ch = 2 nm) due to the enhanced quantum confinement effect. This finding is similar to the layer-dependent bandgap changes observed in 2D materials, revealing the quasi-2D feature of the ultrathin In 2 O 3 films [19] . Fig. 1: Device structures and high-resolution transmission electron microscopy (HRTEM) images of atomic layer deposition (ALD) deposited In 2 O 3 transistors. a Schematic of a 2 nm In 2 O 3 transistor. The inset shows the HRTEM image of the ALD-deposited ultrathin In 2 O 3 films. The scale bar is 5 nm. b Tauc plot of the In 2 O 3 films as a function of film thickness. The fitting of the curve is done based on the Tauc model (α: absorption coefficient; h: Planck’s constant; ν: frequency of vibration). c Transfer curves of 2 nm In 2 O 3 transistors with channel width/length of 10/2 µm and annealed under N 2 and O 2 for 30 min at 150 °C. Note that the amounts of threshold voltage ( V T ) shifts are saturated after 30 minutes ( I D : drain current; V D : drain voltage; V G : gate voltage). Full size image Figure 1c shows the transfer characteristics ( I D – V G ) of 2 nm In 2 O 3 transistors annealed at 200 °C in O 2 and N 2 environments. The transfer characteristics ( I D – V G ) of In 2 O 3 below 2 nm is shown in Supplementary Fig. 5 and saturation behavior ( I D – V D ) is shown in Supplementary Fig. 6 . O 2 and N 2 annealing lead to V T shifts to +6 V and −20 V, respectively; both show effective tuning of V T after 30 min of annealing (the V T extraction method is described in the “Methods” section). While the traditional annealing method can effectively tune the V T of In 2 O 3 transistors, precise control of V T over the tuning range is difficult. 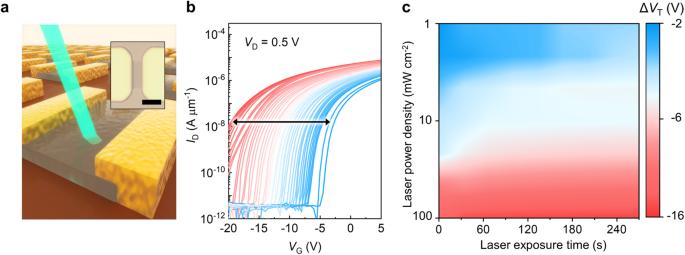Fig. 2:VTtuning in ultrathin In2O3transistors via ultraviolet (UV) exposure. aA schematic ofVTtuning in ultrathin In2O3transistors through UV exposure combined with thermal annealing; the inset is the microscopic image of the transistor with a scale bar of 5 µm.bTransfer curves of 2 nm In2O3transistors with channel width/length of 10/2 µm after post treatments. The arrow represents the transition of transfer curves with UV light exposure (red lines) and O2annealing (blue lines) (ID: drain current;VD: drain voltage;VG: gate voltage).cA contour plot ofVTshifts as a function of UV exposure time and power density. Devices were annealed at 150 °C in O2for 30 min to reset theVTbefore each UV exposure measurement. The absorbed power density increasing from 1\(\times\)106mW cm−2to 1\(\times\)108mW cm−2for exposure times from 30 s to 300 s under 365 nm laser illumination. The measurement time interval is 30 s and the transfer characteristics of the device are immediately measured (<5 s) after UV illumination. The plot consists of 7 different power densities and 10 different exposure times. Figure 2a illustrates the proposed approach to achieve fine-tuning of V T in ultrathin In 2 O 3 transistors. The device is first subjected to O 2 annealing, which shifts the V T to +6 V. Subsequent UV irradiation (365 nm) on In 2 O 3 transistors shifts the V T to the negative values (Fig. 2b ), where the magnitude of V T shifts depends on the exposure time, incident power density and wavelength (Fig. 2c and Supplementary Figs. 7 and 8 ). Note that UV exposure causes an accumulation of V T shift, leading to a saturation point of −15 V with a tuning resolution of 0.05 V within a tunable window Δ V T of 21 V (Supplementary Fig. 9 ). To verify reproducibility of our approach, we tested devices with identical fabrication processes but different metal contacts (Pd, Pt) and substrates (10 nm HfO 2 as the gate dielectric). All results exhibited consistent trends, regardless of substrate and metal contacts. (Supplementary Fig. 10 ). Importantly, the V T modulation using the proposed approach is reversible. UV-exposed In 2 O 3 transistors with negative V T can be reset to have a value of 5 V after O 2 annealing. 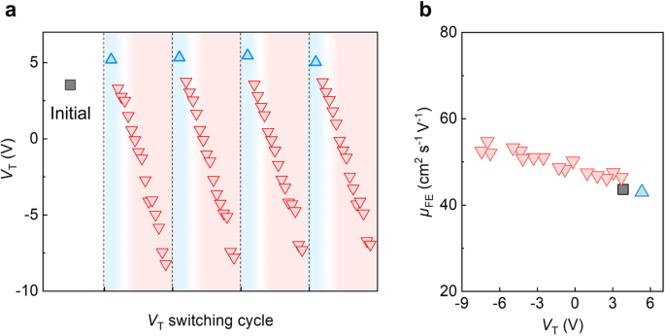Fig. 3: Reversibility ofVTtuning in ultrathin In2O3transistors. aVTof a 2 nm In2O3transistor with channel width/length of 10/2 µm during multiple O2annealing and UV exposure cycles. In2O3transistors are thermally annealed under O2for 30 min, followed by UV illumination under a power density of 1 mW cm−2. The blue triangles are theVTafter O2annealing. The red triangles are theVTafter UV exposure. The dashed lines separate different switching cycle and the shaded areas represent the treatments (blue: O2annealing; red: UV exposure).bThe field effect mobility (\({\mu }_{{FE}}\)) of ultrathin In2O3transistors as a function ofVTtuned by the proposed method. Figure 3a shows repeated V T modulation achieved by multiple O 2 annealing-UV exposure cycles. The field effect mobility ( \({\mu }_{{FE}}\) ) of the transistors is maintained at 49 ± 5 cm 2 V –1 s –1 , indicating that the properties of the In 2 O 3 transistors are not significantly affected by the tuning V T processes (Fig. 3b ). Additionally, we also conduct the bias stress experiment to investigate behavior and reliability of transistors under different bias conditions after the treatment of O 2 annealing and UV exposure (Supplementary Fig. 11 ). A gate voltage was applied at ±15 V for 1000 s, with both source and drain grounded. The transfer characteristics of the device are immediately measured (<1 s) after bias stress. Furthermore, to evaluate the potential damage caused by laser exposure, we performed finite element simulations to analyze the temperature changes. The results indicate only a slight increase in temperature at the applied incident power densities (Supplementary Fig. 12 ). Fig. 2: V T tuning in ultrathin In 2 O 3 transistors via ultraviolet (UV) exposure. a A schematic of V T tuning in ultrathin In 2 O 3 transistors through UV exposure combined with thermal annealing; the inset is the microscopic image of the transistor with a scale bar of 5 µm. b Transfer curves of 2 nm In 2 O 3 transistors with channel width/length of 10/2 µm after post treatments. The arrow represents the transition of transfer curves with UV light exposure (red lines) and O 2 annealing (blue lines) ( I D : drain current; V D : drain voltage; V G : gate voltage). c A contour plot of V T shifts as a function of UV exposure time and power density. Devices were annealed at 150 °C in O 2 for 30 min to reset the V T before each UV exposure measurement. The absorbed power density increasing from 1 \(\times\) 10 6 mW cm −2 to 1 \(\times\) 10 8 mW cm −2 for exposure times from 30 s to 300 s under 365 nm laser illumination. The measurement time interval is 30 s and the transfer characteristics of the device are immediately measured (<5 s) after UV illumination. The plot consists of 7 different power densities and 10 different exposure times. Full size image Fig. 3: Reversibility of V T tuning in ultrathin In 2 O 3 transistors. a V T of a 2 nm In 2 O 3 transistor with channel width/length of 10/2 µm during multiple O 2 annealing and UV exposure cycles. In 2 O 3 transistors are thermally annealed under O 2 for 30 min, followed by UV illumination under a power density of 1 mW cm −2 . The blue triangles are the V T after O 2 annealing. The red triangles are the V T after UV exposure. The dashed lines separate different switching cycle and the shaded areas represent the treatments (blue: O 2 annealing; red: UV exposure). b The field effect mobility ( \({\mu }_{{FE}}\) ) of ultrathin In 2 O 3 transistors as a function of V T tuned by the proposed method. Full size image The size of the tunable window Δ V T is dependent on the thickness of the In 2 O 3 , as shown in Fig. 4a, b ( V T shift as a function of channel length is shown in Supplementary Fig. 13 ). In 2 O 3 with a thickness of 4 nm shows the largest tunable window, whereas In 2 O 3 with a thickness of 2 nm is capable of being tuned between the enhancement mode ( V T > 0 V) and the depletion mode ( V T < 0 V). The offsets of tunable window for different thickness can be explained by the quantum confinement effect on the trap-neutral level model [19] . Fermi level is located deeply inside the conduction band for thicker In 2 O 3 and aligns within the bandgap for thinner In 2 O 3 as the bandgap is enlarged due to the enhanced quantum confinement effect. Fig. 4: Tunable V T windows and benchmarks of In 2 O 3 transistors versus other ultrathin transistors. a The range of the tunable window of In 2 O 3 transistors with various In 2 O 3 thicknesses, channel width/length of 10/2 µm. b The range of V T after treatment. c Benchmark of sheet carrier density ( n 2D ) for different classes of ultrathin semiconductors with different thicknesses [20] , [21] , [22] , [23] , [24] , [25] , [26] , [27] , [28] , [29] , [30] , calculated using both the Drude model and the parallel-plate capacitor model. The shaded areas represent different classes of materials (red: In 2 O 3 ; purple: monolayer 2D materials). d The Δ n 2D for different classes of ultrathin semiconductors based on capacitively charged structures. Shaded area represents different material categories (red: In 2 O 3 ; green: ferroelectric memories; yellow: flash memories). Full size image To further quantify the V T shift, we extract 2D carrier density ( \({n}_{2D}\) ) using the Drude model \({n}_{2D}={I}_{D}L/({qW}{V}_{D}{\mu }_{{FE}})\) , where q is the electron charge, I D is the source-drain current at zero gate voltage, V D is the source-drain voltage, and μ is the field effect carrier mobility. Based on the Drude model, we benchmark our method against other V T tuning methods used in different classes of ultrathin semiconductors. 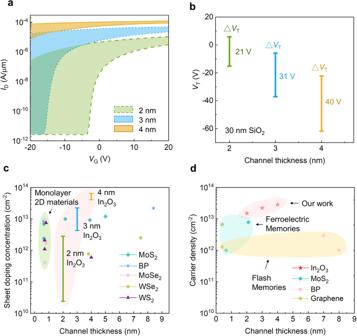Fig. 4: TunableVTwindows and benchmarks of In2O3transistors versus other ultrathin transistors. aThe range of the tunable window of In2O3transistors with various In2O3thicknesses, channel width/length of 10/2 µm.bThe range ofVTafter treatment.cBenchmark of sheet carrier density (n2D) for different classes of ultrathin semiconductors with different thicknesses20,21,22,23,24,25,26,27,28,29,30, calculated using both the Drude model and the parallel-plate capacitor model. The shaded areas represent different classes of materials (red: In2O3; purple: monolayer 2D materials).dThe Δn2Dfor different classes of ultrathin semiconductors based on capacitively charged structures. Shaded area represents different material categories (red: In2O3; green: ferroelectric memories; yellow: flash memories). Figure 4c shows the n 2D of 2D semiconductors modulated by various chemical doping schemes [20] , [21] , [22] , [23] , [24] , [25] , [26] , [27] , [28] , [29] , [30] , which ranges from 10 12 to 10 13 cm −2 depending on the doping methods and materials (details in Supplementary Table 2 ). The tunable ranges of n 2D achieved in In 2 O 3 transistors vary from 10 10 cm −2 to 10 13 cm −2 depending on the thickness. 2 nm In 2 O 3 exhibits the widest n 2D tunable window (2 \(\times\) 10 10 cm −2 to 2 \(\times\) 10 12 cm −2 ), indicating the proposed method is competitive among various 2D doping techniques. The proposed methods offer a comparable effect to chemical doping, while providing the advantages of reversibility and area selectivity. In contrast to the substantial challenges associated with chemical doping in 2D materials, our method showcases the ease of achieving effective carrier concentration tuning in ultrathin In 2 O 3 . Moreover, our approach minimizes fabrication processes, thereby enhancing its potential for seamless integration in BEOL applications. Another commonly used approach to control the V T of a transistor is through device design, usually done by inserting a layer that can be capacitively charged. For instance, flash memories store charge in a charge-trapping layer to modulate V T through the trapping and de-trapping process. Similarly, ferroelectrics modulate V T by controlling the polarization of a ferroelectric layer. The density of stored charge carriers n 2D is around 10 12 cm −2 to 10 13 cm −2 for graphene and related 2D materials-based flash memories and ferroelectric memories. The Δ n 2D for In 2 O 3 extracted by the parallel-plate capacitor model (1.5 \(\times\) 10 13 , 2.3 \(\times\) 10 13 and 2.8 \(\times\) 10 13 cm −2 for 2, 3 and 4 nm, respectively) is of the same order as flash memories and ferroelectric memories without extra gates (Fig. 4d ) [9] , [31] , [32] , [33] , [34] , [35] . The details of 2D-based charge-storing schemes are summarized in Supplementary Table 3 . Compared to other 2D doping and capacitively charged techniques, the proposed method demonstrates a more effective way to largely tune the carrier density in In 2 O 3 transistors, enabling In 2 O 3 transistors for innovative circuit and memory applications. We conducted cyclically annealing between N 2 and O 2 environments to investigate the mechanism (Supplementary Fig. 14 ). The results demonstrate that the V T shift by N 2 and O 2 annealing is reversible, similar to the reversibility observed in UV exposure and O 2 annealing processes. This result implies that the mechanisms underlying these two approaches may be identical. It is known that electronic properties of amorphous In 2 O 3 can be altered by oxygen-related defects such as oxygen vacancies and oxygen adatoms on the surface [36] . Oxygen vacancies act as shallow donors and contribute to the spontaneous n-type conductivity of the In 2 O 3 (the shallow donor level is observed in scanning tunneling microscopy (STS) shown in Supplementary Fig. 15 ). Oxygen adatoms, on the other hand, act as acceptor-like traps that counter-dope the n-type OS. Annealing in oxygen-rich or oxygen-scarce (N 2 or vacuum) environments causes a rebalance of physically adsorbed oxygen adatoms, leading to positive and negative V T shifts, respectively. Furthermore, exposure to UV light generates holes that neutralize the negatively charged oxygen adatoms, resulting in their detachment and a decrease in the V T . This proposed mechanism is supported by the measurement of V T retention in different atmospheres, as shown in Supplementary Fig. 16 . Additionally, the V T exhibits almost no change over time in an ultra-high vacuum environment (10 −9 torr), which further highlights the crucial role of oxygen adatoms in this process. The results suggest that the stability could be improved by implementing effective isolation or passivation to minimize the exposure of In 2 O 3 to the atmosphere. Demonstration of depletion-load inverter and multi-step logic The proposed method allows for precise control of V T , making it useful for advanced low-power circuits [37] . Here, we demonstrate a depletion-load inverter by adjusting the V T of the selected In 2 O 3 transistors in a circuit, achieved by employing a micro-laser system that can focus UV exposure selectively on In 2 O 3 transistors (details in “Methods”). 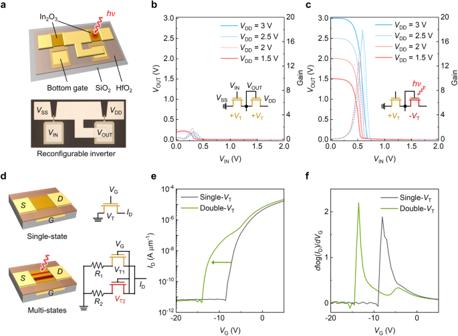Fig. 5: Applications of ultrathin In2O3transistor with laser exposure. aA schematic and optical microscope image of In2O3inverter (h: Planck’s constant;ν: frequency of vibration;VDD: drain voltage;VSS: source voltage;VIN: input voltage;VOUT: output voltage).bThe voltage transfer characteristics of 2 nm In2O3inverter with channel width/length of 10/2 µm before UV laser illumination.cThe voltage transfer characteristics of In2O3inverter of 2 nm In2O3inverter with channel width/length of 10/2 µm after UV laser illumination.dA schematic of ultrathin In2O3transistor with multi-state logic function (VG: gate voltage;ID: drain current;R1: resistance of first channel;R2: resistance of second channel;VT1: threshold voltage of first channel;VT2: threshold voltage of second channel).e, The transfer characteristics of In2O3transistor with UV laser illumination on the specific area.fThe transfer characteristics with the first-order derivative of log(ID) frome. 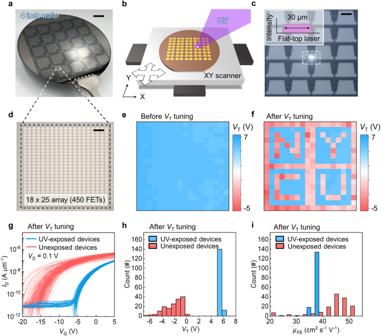Fig. 6: Large-areaVTmodulation. aAn image of ultrathin In2O3transistor arrays on a 4-inch wafer. The scale bar is 1 cm.bSchematics of the automated laser illumination system used forVTmodulation.cAn optical microscope image of UV laser exposure on the designated channel area. The inset is the illustration of flat-top laser beams. The scale bar is 50 µm.dAn optical microscope image of the basic array unit on 4-inch wafer consisted of an 18\(\,\times \,\)25 array (450 transistors). The scale bar is 200 µm.eA contour plot showing theVTof the transistors in the array beforeVTtuning.fA contour plot showing theVTof the transistors in the array afterVTtuning.gThe transfer curves of the devices with channel width/length of 10/2 µm in the array afterVTtuning (red line: UV exposed areas; blue line: unexposed area).hThe histogram ofVTof the devices in the array afterVTtuning.iThe histogram of\({\mu }_{{FE}}\)of the devices in the array afterVTtuning. Figure 5a illustrates the layout of an inverter circuit with two n-type In 2 O 3 transistors connected by local bottom gates. Both transistors are set to enhancement mode via O 2 annealing, resulting in a V T shift to +5 V. When V DD is applied, V OUT is limited as the channel resistance of the load transistor is large, resulting in a small gain of 2 for V DD = 3 V (Fig. 5b ). After exposing the load transistor to UV light, tuning the selected transistor to depletion mode, the inverter becomes a depletion-load inverter with an enhanced gain of 18 (Fig. 5c ). Note that the depletion load inverter serves as a proof of concept for our proposed technology. Integrating a complementary MOS configuration has the potential to further optimize the performance of inverters, resulting in reduced power consumption and improved spatial advantages. The functionality of the circuit is activated via the proposed method with local V T tunability, giving a higher degree of freedom to design and calibrate the circuit even after fabrication. Fig. 5: Applications of ultrathin In 2 O 3 transistor with laser exposure. a A schematic and optical microscope image of In 2 O 3 inverter ( h : Planck’s constant; ν : frequency of vibration; V DD : drain voltage; V SS : source voltage; V IN : input voltage; V OUT : output voltage). b The voltage transfer characteristics of 2 nm In 2 O 3 inverter with channel width/length of 10/2 µm before UV laser illumination. c The voltage transfer characteristics of In 2 O 3 inverter of 2 nm In 2 O 3 inverter with channel width/length of 10/2 µm after UV laser illumination. d A schematic of ultrathin In 2 O 3 transistor with multi-state logic function ( V G : gate voltage; I D : drain current; R 1 : resistance of first channel; R 2 : resistance of second channel; V T1 : threshold voltage of first channel; V T2 : threshold voltage of second channel). e , The transfer characteristics of In 2 O 3 transistor with UV laser illumination on the specific area. f The transfer characteristics with the first-order derivative of log( I D ) from e . Full size image The ability to locally adjust the V T with high spatial resolution in In 2 O 3 transistors allows for creating non-uniform V T patterns in the channel and enables new functions. We demonstrate that a reconfigurable In 2 O 3 transistor can switch between binary and multi-state logic without the need for multiple gates [38] or heterojunctions [39] . Figure 5d illustrates a transistor with uniform V T along the channel detailed in Supplementary Fig. 17 . After UV exposure on the selected area, non-uniform V T pattern forms on the channel. The equivalent circuit configuration changes depending on the scanning pathways, consisting of parallel resistors and transistors with different V T depending on the exposure time. As a result, a single swing in transfer characteristics turns to double-swing characteristics (Fig. 5e, f ), increasing the information capacity of a single transistor. The demonstration of an In 2 O 3 -based multi-state logic device introduces an alternative strategy to design reconfigurable multifunctional logic circuits and has the potential for neuromorphic applications (Supplementary Fig. 18 ) [40] , [41] . Wafer-scale V T modulation To further demonstrate the practicability of our technique, we fabricated In 2 O 3 transistors on a 4-inch wafer (Fig. 6a ) and employed an automated laser illumination system (Laser Lift-Off System; K-JET LASER TEK Inc.) for large-scale V T tuning (Fig. 6b ). The system allows for precise alignment to direct focused flat-top illumination onto selected devices, enabling localized V T modulation (Fig. 6c , Supplementary Movie 1 and tool details in Methods). We demonstrate the scalability by tuning V T for 450 transistors in an 18 \(\times \) 25 array (Fig. 6d ). The initial V T was set to ~7 V through O 2 annealing for all transistors (Fig. 6e ), and the V T of the laser-exposed transistors were tuned to negative values (Fig. 6f ). The transfer curves after V T modulation were shown in Fig. 6g , demonstrating the consistency of the proposed approach. The V T of unexposed transistors remained the same after the large-area tuning, as shown in Fig. 6h . The \({\mu }_{{FE}}\) distribution shows that the mobility increases slightly after UV exposure (Fig. 6i ), in agreement with previous results. Note that the device-to-device variation, induced by the variation in film quality across the wafer, may potentially be mitigated through the utilization of industrial-level ALD tools. Furthermore, the V T tuning precision could be improved by the incorporation of patterned photomasks. This demonstration not only shows capability of wafer-scale fabrication and V T tuning on multiple transistors, but also opens up possibilities for enhancing circuit functionality beyond V T adjustment. Fig. 6: Large-area V T modulation. a An image of ultrathin In 2 O 3 transistor arrays on a 4-inch wafer. The scale bar is 1 cm. b Schematics of the automated laser illumination system used for V T modulation. c An optical microscope image of UV laser exposure on the designated channel area. The inset is the illustration of flat-top laser beams. The scale bar is 50 µm. d An optical microscope image of the basic array unit on 4-inch wafer consisted of an 18 \(\,\times \,\) 25 array (450 transistors ) . The scale bar is 200 µm. e A contour plot showing the V T of the transistors in the array before V T tuning. f A contour plot showing the V T of the transistors in the array after V T tuning. g The transfer curves of the devices with channel width/length of 10/2 µm in the array after V T tuning (red line: UV exposed areas; blue line: unexposed area). h The histogram of V T of the devices in the array after V T tuning. i The histogram of \({\mu }_{{FE}}\) of the devices in the array after V T tuning. Full size image In summary, we demonstrate the wide-range V T tunability in ultrathin In 2 O 3 using an optical–thermal method. This approach is comparable to doping and capacitively charged techniques used in other ultrathin semiconductors and avoids the need for external dopants and complex processes. Our demonstration of a depletion-load inverter suggests that this V T tuning method has the potential to enable new functionalities in combinational logic circuits. Additionally, we have demonstrated a single device with multi-state logic function, which opens up new possibilities for the design of multifunctional logic circuits and non-von Neumann computing. Moreover, we conducted large-scale V T modulation using an industry-level tool to highlight the practical applicability of this method alongside individual device testing. Device fabrication The device fabrication started with a standard wet and dry pre-clean of 300 mm Si substrate. The highly phosphorus-doped Si, which carrier density is over 10 21 cm −3 , was grown on Si substrate as a global back-gate. Then, 30 nm SiO 2 was deposited by ALD at 260 °C with (H 2 Si[N(C 2 H 5 ) 2 ] 2 ) as the precursor. Afterwards, In 2 O 3 thin films with different thicknesses were deposited by ALD at 200 °C using (CH 3 ) 3 In (TMIn) and O 3 as indium (In) and oxygen (O) precursors. The active areas of In 2 O 3 were defined by lithography with HCl etching with the channel width/length of 10/2 µm. Standard lithography patterning and lift-off procedures were performed to contact the In 2 O 3 thin films with metal electrodes. 40 nm Ni was deposited by e-beam evaporation on In 2 O 3 to serve as source/drain ohmic contacts. Inverter fabrication The inverter fabrication started with a standard wet and dry pre-clean of 250 mm Si with a 50 nm SiO 2 substrate. Then, the local back gate of 40 nm Ni was deposited by e-beam evaporation. Afterwards, 6 nm HfO 2 was deposited by ALD at 250 °C with TDMAHf as a precursor for 70 cycles. After the gate dielectric deposition, 2 nm In 2 O 3 thin films were deposited by ALD at 200 °C using (CH 3 ) 3 In (TMIn) and O 3 as In and O precursors. The active areas of In 2 O 3 were defined by lithography with HCl etching for 5 s. Then, the contact holes were patterned by standard lithography, followed by BOE etching for 5 min. Finally, a Ni (40 nm) film was deposited by e-beam evaporation to serve as source/drain ohmic contacts and metal line interconnections. Device characterization As-grown In 2 O 3 was then measured for thickness using a transmission electron microscope (TEM). A focused ion beam (FIB) system (Auriga, Carl Zeiss) was used to fabricate the cross-sectional specimen, which was then examined by a TEM (none-Cs Metrios). The electronic characteristics were measured by an Agilent B2902B source. The \({\mu }_{{FE}}\) and V T of ultrathin In 2 O 3 transistors were determined in linear regime using conventional MOSFET equation for \({V}_{D}\ll {V}_{G}-{V}_{T}\) : \({I}_{D}=\frac{W}{L}{\mu }_{{FE}}{C}_{{OX}}({V}_{G}-{V}_{T}){V}_{D}\) , where C OX is the oxide capacitance. The result of \({\mu }_{{FE}}\) can be obtained from \({\mu }_{{FE}}=\frac{L{g}_{m}}{W{C}_{{OX}}{V}_{D}} \) , where g m is maximum transconductance. The resulted V T was determined by linear extrapolation, which was conducted by plotting I D versus V G , extrapolating from maximum transconductance ( g m ) to I D = 0 and adding V D /2 to obtain the intercept at V G axis. Laser exposure The 365 and 532 nm laser beams were generated by diode lasers (RGB Laser systems, Lambda Beam). The laser light passes through a shutter (NM Laser Product, LST-5VDC) to control the laser exposure time. Following the shutter, an ND filter was used to control the laser incident power. After that, the laser beam (365, 532 nm) was focused on the device through a fixed optical path using a ×50 objective lens (OLYMPUS, LMPlanFL N ×50, NA  = 0.5) with a laser spot diameter of ~10 μm. Meanwhile, the absorbed power was measured by a power meter which comprised a detector (Thorlab, S120VC) and a meter (Thorlab, PM100D). Thermal annealing The fabricated devices were placed in a customized chamber with two gas inlets. Then, the devices were annealed in O 2 and N 2 with 1 liter per minute gas flow for 30 min at 150 °C. The pressure was kept at about 1 atm. Absorption spectra The In 2 O 3 films were deposited on a 200 μm-thick glass substrate following the same ALD process as mentioned before. An ellipsometer determined the thickness of In 2 O 3 films for absorption measurement. A Hitachi U-4100 spectrophotometer was used to investigate the transmittance of samples between the 300 and 700 nm range with an integrating sphere. Absorptance of the films was calculated using the relation A = 100 − ( T + R ). Wafer-scale V T modulation Wafer-scale V T modulation was achieved using an automatic laser illumination tool (Laser Lift-Off System; K-JET LASER TEK Inc.). The laser spot size and shape can be customized by a mask based on our specific needs, allowing for arbitrary adjustments. The laser intensity is uniformly distributed across the entire exposure area (20 µm \(\times \) 1 µm for this study), commonly known as flat-top beams, achieved via applying a mask on the optical path to ensure consistent laser exposure within the targeted region. Laser pulses with energy of 0.0015 J/cm 2 , a wavelength of 365 nm, and a pulse width of 26 ns were directed onto the desired regions or devices. The scanning rate is ~1 ms/transistor.